Concomitant Notch activation and p53 deletion trigger epithelial-to-mesenchymal transition and metastasis in mouse gut Epithelial-to-mesenchymal transition-like (EMT-like) is a critical process allowing initiation of metastases during tumour progression. Here, to investigate its role in intestinal cancer, we combine computational network-based and experimental approaches to create a mouse model with high metastatic potential. Construction and analysis of this network map depicting molecular mechanisms of EMT regulation based on the literature suggests that Notch activation and p53 deletion have a synergistic effect in activating EMT-like processes. To confirm this prediction, we generate transgenic mice by conditionally activating the Notch1 receptor and deleting p53 in the digestive epithelium ( NICD/p53 −/− ). These mice develop metastatic tumours with high penetrance. Using GFP lineage tracing, we identify single malignant cells with mesenchymal features in primary and metastatic tumours in vivo . The development of such a model that recapitulates the cellular features observed in invasive human colorectal tumours is appealing for innovative drug discovery. Tumour metastasis, the main cause of death in cancer patients, is a multi-step process in which tumour cells exit their original tissue, migrate to distant locations and survive in new microenvironments [1] , [2] . This plasticity results from the accumulation of genetic mutations, epigenetic modifications and involves a reversible biological process, the epithelial-to-mesenchymal transition-like (EMT-like) [3] . The EMT is initiated by key transcription factors, including SNAIL, SLUG, TWIST, ZEB1 and ZEB2 regulating downstream targets transcription. This leads to E-cadherin (ECAD) loss [4] , [5] , epithelial cells cytoskeleton disorganization, cell adhesion complexes loss and elongated fibroblast phenotype acquisition accompanied by vimentin, fibronectin or α-smooth muscle actin (α-SMA) expression [6] . EMT is important during embryonic development for the formation of body plan and the differentiation of tissues and organs [7] . Data from human solid cancers, cell culture and xenograft systems show that an EMT-like phenotype leads to poor clinical outcomes and enhances cell invasiveness and migration [8] , [9] , [10] , [11] . A spontaneous squamous cell carcinoma mouse model has demonstrated the requirement of EMT-like in tumour metastasis in vivo [12] . However, while the significance of the EMT-like process during tumour progression is accepted, the full demonstration of its existence in cancer is still debated owing to the difficulty in distinguishing normal resident stromal cells from pathological mesenchymal cells originating from malignant epithelial cells through an EMT-like process [3] . In colorectal cancer (CRC), 25% of patients present with overt metastases; additional 25–35% of patients will develop metastases during disease progression [13] , thereby making CRC an appropriate model to study EMT-like processes. Despite the existence of knowledge of the mutational landscape initiating CRC, the mechanisms of disease progression related to EMT are poorly understood. To study the role of EMT in disease progression, a lineage tracing strategy with tissue specificity is needed. Such approach has been applied to describe EMT-like phenotype in pancreatic cancer [14] . However, epithelial lineage tracing experiments have been performed neither in a mouse model of metastatic colon cancer with liver metastases [15] nor in other metastatic models with activated KRAS and TGFBR2 deletion [16] or activated KRAS and PTEN loss [17] . Therefore, the earliest events preceding the appearance of metastases could not be captured in these mouse models, thus leaving an open question about direct involvement of such mutations in EMT-like induction. The aim of our study was to generate a mouse model developing invasive intestinal cancer with high penetrance, allowing in vivo dissection of molecular mechanisms in EMT and metastasis. We use a computational biology approach for rationalizing the choice of such a combination of molecular targets that would trigger the EMT-like and metastatic phenotype. Systematic literature study allows assembling EMT regulation signalling network followed by network structural analysis. It is predicted that p53 loss and Notch activation should have synergistic effect on the EMT-like phenotype induction. To validate this hypothesis, we create a transgenic mouse model expressing a constitutively active Notch1 receptor in a p53 -deleted background, specifically in the digestive epithelium. Importantly, green fluorescent protein (GFP) expression linked to the Notch1 receptor activation allows lineage tracing of epithelial tumour cells during cancer progression and invasion. These mice develop digestive tumours with dissemination of EMT-like epithelial malignant cells to the lymph nodes, liver and peritoneum and generation of distant metastases. These transgenic mice represent an appropriate in vivo model to study the EMT-like process of malignant cells from the primary tumour to metastasis. We confirm the presence of EMT-like cells expressing the EMT-inducer ZEB1 but not the epithelial marker ECAD in human invasive primary CRC and metastases. Signalling network reconstruction and analysis The reactivation of developmental mechanisms in tumour cells is believed to govern the EMT-like processes that lead to cell dissemination [3] . In order to achieve early EMT-like with dissemination in multiple organs, we have explored early inducers of the EMT programme. Since the single transgenic mouse mutants currently described never developed distant metastasis, we hypothesized that reactivation of EMT programme requires affecting activity of several genes that can interact in a synergic manner. To identify combination of genes that could be responsible for the induction of EMT-like phenotype, we systematically revised the existing literature and pathway databases for mechanisms inducing EMT. This information was gathered together into a comprehensive map of signalling involved in EMT regulation (see Methods section). The map depicts the mechanisms of EMT regulation by p53, Notch, AKT and MAPK (downstream signalling of Ras), Wnt, transforming growth factor-β signalling and miRNAs. Important regulators of differentiation, apoptosis and proliferation have been included to depict the crosstalk between these regulatory circuits and their competition with the EMT programme ( Supplementary Fig. 1A ). Interactive online version of the map accompanied by detailed description of the molecular mechanisms and the comprehensive list of references can be found at https://navicell.curie.fr/pages/signalling_network_emt_regulation_description.html . We performed structural analysis and simplification of the EMT network ( Supplementary Fig. 1B,C ; see Methods section) that highlighted the following EMT network organization principles, which is in agreement with current EMT understanding: (1) five EMT transcription factors SNAIL, SLUG, TWIST, ZEB1 and ZEB2 that have partially overlapping sets of downstream target genes can activate the EMT-like programme [18] . (2) These key EMT transcription factors are under control of several upstream mechanisms: they are directly induced at the transcriptional level by the activated form of Notch, NICD [19] , but are downregulated at the translational level by several miRNAs (namely, mir200, mir34, mir203 and mir192) that are under transcriptional control of p53 family genes [20] . Interestingly, some key EMT transcription factors can inhibit microRNAs, in this way sustaining their own activation [21] , [22] . (3) According to the network structure, all five key EMT transcription factors should be activated ensuring simultaneous activation of EMT-like programme genes and downregulating miRNAs. In addition, the EMT key inducers also inhibit apoptosis [18] and reduce proliferation [23] . (4) The activity of Wnt pathway is stimulated by transcriptional activation of the gene coding for β-catenin protein by Notch-induced TWIST or SNAI1 (ref. 24 ). The Wnt pathway, in turn, can induce the expression of Notch pathway factors, creating a positive feedback loop [25] . In agreement with other studies, the Wnt pathway does not directly induce EMT, but helps to maintain it [24] . (5) Components of the Wnt and Notch pathways are negatively regulated by miRNAs induced by the p53 family (p53, p63 and p73). The balance between the effect of positive (Notch and Wnt) and negative (p53, p63 and p73 mediated by miRNAs) regulatory circuits on EMT inducers dictates the possibility of EMT phenotype. In order to clarify the interplay between Wnt, Notch and p53 pathways, we performed network complexity reduction up to core regulators of EMT, apoptosis and proliferation that were preserved through all levels of reduction ( Supplementary Fig. 1B,C ; see Methods section). The reduced network has been used for comparison between the wild-type (WT) cells and all possible combinations of single and double mutants for Wnt pathway, Notch and p53 for achieving EMT-like phenotype. Network analysis shows that the loss of function of p53 alone can be compensated by p63/p73, inducing the same set of microRNAs and, thus, inhibiting EMT. Activated p63/p73 may induce apoptosis in the rare situations when p53 −/− cells start to undergo EMT ( Fig. 1 and Supplementary Fig. 2 ). This model may explain the non-invasive sporadic tumours in p53 −/− mice [26] . This prediction is also supported by latest observation in the Braf V637E , where p53 does not affect early stages of Braf V637E -induced tumorigenesis but has an important role in invasiveness prevention [27] . 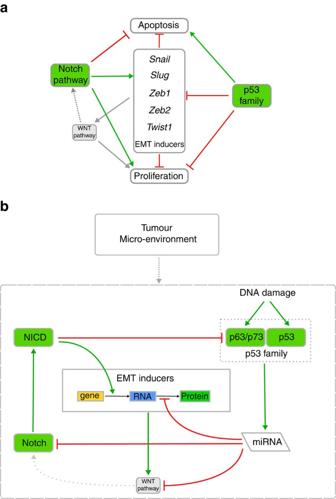Figure 1: A hypothesis on Notch–p53 and Wnt interplay derived from signalling network analysis. Green and grey arrows indicate an activating effect, red arrows depict an inhibiting effect and dotted line indicates an indirect effect. (a) Schematic view of three signalling pathways (Wnt, Notch and p53) and the phenotypes of apoptosis, proliferation and EMT induction, showing crosstalk between each other. (b) Schematic view at a molecular level showing the involvement of Notch and Wnt pathways, p53 family and microRNAs in activating EMT inducers. The p53 family members (p53, p63 and p73) can be activated by DNA damage and can induce transcription of miRNAs (for example, miR34, miR200 and miR203). These miRNAs target mRNAs coding for β-catenin(Wnt pathway),Notchand the EMT inducers (Snail, Twist, Slug, Zeb1andZeb2). Those EMT inducers activate the Wnt pathway that, in turn, activates the Notch pathway, resulting in the activation of Notch (NICD). NICD activates the gene expression of EMT inducers, but can also inhibit transcription of p63 and p73, but not p53. Various signals from tumour microenvironment as extracellular matrix (ECM) components, hormones, growth factors, inflammatory factors and so on (collectively denoted as ‘Tumour microenvironment’ node) can sensitize the activation of EMT programme only in those cells that are in contact with microenvironmental signals. Figure 1: A hypothesis on Notch–p53 and Wnt interplay derived from signalling network analysis. Green and grey arrows indicate an activating effect, red arrows depict an inhibiting effect and dotted line indicates an indirect effect. ( a ) Schematic view of three signalling pathways (Wnt, Notch and p53) and the phenotypes of apoptosis, proliferation and EMT induction, showing crosstalk between each other. ( b ) Schematic view at a molecular level showing the involvement of Notch and Wnt pathways, p53 family and microRNAs in activating EMT inducers. The p53 family members (p53, p63 and p73) can be activated by DNA damage and can induce transcription of miRNAs (for example, miR34, miR200 and miR203). These miRNAs target mRNAs coding for β -catenin (Wnt pathway), Notch and the EMT inducers ( Snail, Twist, Slug, Zeb1 and Zeb2 ). Those EMT inducers activate the Wnt pathway that, in turn, activates the Notch pathway, resulting in the activation of Notch (NICD). NICD activates the gene expression of EMT inducers, but can also inhibit transcription of p63 and p73, but not p53. Various signals from tumour microenvironment as extracellular matrix (ECM) components, hormones, growth factors, inflammatory factors and so on (collectively denoted as ‘Tumour microenvironment’ node) can sensitize the activation of EMT programme only in those cells that are in contact with microenvironmental signals. Full size image In the Notch gain-of-function mutants, transcriptional activation of EMT inducers may be counterbalanced by p53-activated microRNAs at the translational level, possibly explaining the lack of invasive tumours in the NICD mice [28] , [29] ( Fig. 1 and Supplementary Fig. 2 ). In Apc heterozygous loss-of-function mutants (considered as Apc −/− in this study), increased activation of the Wnt pathway might lead to activation of the Notch pathway. However, the p53/63/73 family controls Wnt and Notch signals via microRNAs. Therefore, an EMT phenotype is not predicted in this mutant, recapitulating the experimental results [30] . We show that an EMT-like phenotype cannot result from any of the single mutants; therefore, we investigated this process in double mutants. We predict that in Apc −/− /p53 −/− double mutant, Wnt activation does not induce EMT, because p63/p73 induced microRNAs can still inhibit the Wnt and Notch pathway ( Fig. 1 and Supplementary Fig. 2 ). When Notch is activated in an Apc −/− background, cell proliferation is increased as has been observed in the mice models [29] . At the same time, EMT is inhibited by the microRNA expression induced by p53 ( Fig. 1 and Supplementary Fig. 2 ), resulting in non-invasiveness. This explains the observed absence of metastases in NICD/Apc −/− mice [29] . Finally, in NICD/p53 −/− double mutant, other members of p53 family cannot rescue the function of p53 anymore as constitutively activated Notch inhibits the activity of both p63 and p73 (ref. 31 ). NICD activates the transcription of the EMT key inducers and inhibits the production of microRNAs by suppressing p63/p73 in the context of p53 −/− . Notch and p53 have opposite effects on EMT inducers, and overexpression of NICD and knocking-out p53 should have synergetic effect. Furthermore, EMT inducers may activate the Wnt pathway, possibly resulting in a positive feedback loop that will amplify Notch activation and maintain an EMT-like programme. Therefore, our computational analysis of the signalling network leads to the prediction that the simultaneous activation of Notch and loss of p53 can promote an EMT-like phenotype. Development of a conditional mouse model of digestive cancer We generated mutant mice expressing NICD in the intestinal epithelium, in a conditional invalidation of p53 , using villin - CreERT2 tamoxifen-dependent intestine-specific recombination [26] , [32] , [33] . Association of GFP expression with NICD allows tracing of epithelial cells after recombination. We first analysed NICD or p53 −/− single-mutant mice and revealed that neither the loss of p53 nor the activation of Notch alone has an effect in promoting invasive tumours in agreement with the computational predictions and previous data [29] , [34] , [35] . Despite relatively long lifespans, only three animals in each group ( n =20) developed adenocarcinomas after 9 months without metastatic progression ( Fig. 2a,b ). 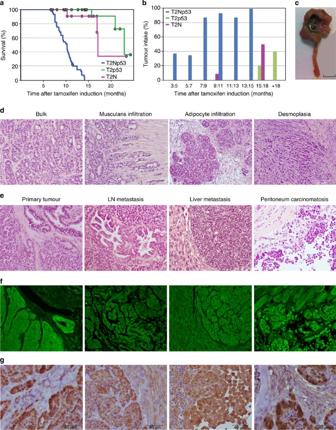Figure 2: Characterization ofNICD/p53−/−primary tumours and metastases. (a) Kaplan–Meier analysis ofNICD/p53−/−mice and their single transgenic littermatesNICD(pink) andp53−/−(green) over a period of 2 years. The triple transgenic mice (blue) are all dead by 15 months with gut adenocarcinoma, whereas control littermates (pink and green) are dying after 15 months. (b) Tumour intake in the intestinal tract ofNICD/p53−/−cohort mice and their relative control littermates at different time points after tamoxifen induction.NICD/p53−/−mice (blue) develop intestinal adenocarcinoma faster and with a higher penetrance than control littermates (pink and green). (c) Macroscopic view of a primary invasive adenocarcinoma located in the jejunum of aNICD/p53−/−mouse. Scale bar, 1 cm. (d) haematoxylin and eosin staining (H&E) staining on paraffin-embedded primary tumour fromNICD/p53−/−mice, representing main features of the tumour. Cancer cells are invading all layers of normal tissue to reach the serosa. We suspect that elongated, single cancer cells are present in desmoplastic areas. Scale bar, 40 μm. (e) H&E and (f) nuclear GFP stainings showing primary tumour, lymph node and liver metastases, and peritoneal carcinomatosis inNICD/p53−/−compound mice. Notice the nonspecific staining due to autofluorescence in the surrounding tumour tissue of lymph node (LN) or liver metastasis and peritoneum carcinomatosis. Scale bars, 40 μm. (g) Immunohistochemical staining of β-catenin showing its nuclear delocalization in cancer cells and its overexpression at the tumour front. Scale bars, 40 μm. Figure 2: Characterization of NICD/p53 −/− primary tumours and metastases. ( a ) Kaplan–Meier analysis of NICD/p53 −/− mice and their single transgenic littermates NICD (pink) and p53 −/− (green) over a period of 2 years. The triple transgenic mice (blue) are all dead by 15 months with gut adenocarcinoma, whereas control littermates (pink and green) are dying after 15 months. ( b ) Tumour intake in the intestinal tract of NICD/p53 −/− cohort mice and their relative control littermates at different time points after tamoxifen induction. NICD/p53 −/− mice (blue) develop intestinal adenocarcinoma faster and with a higher penetrance than control littermates (pink and green). ( c ) Macroscopic view of a primary invasive adenocarcinoma located in the jejunum of a NICD/p53 −/− mouse. Scale bar, 1 cm. ( d ) haematoxylin and eosin staining (H&E) staining on paraffin-embedded primary tumour from NICD/p53 −/− mice, representing main features of the tumour. Cancer cells are invading all layers of normal tissue to reach the serosa. We suspect that elongated, single cancer cells are present in desmoplastic areas. Scale bar, 40 μm. ( e ) H&E and ( f ) nuclear GFP stainings showing primary tumour, lymph node and liver metastases, and peritoneal carcinomatosis in NICD/p53 −/− compound mice. Notice the nonspecific staining due to autofluorescence in the surrounding tumour tissue of lymph node (LN) or liver metastasis and peritoneum carcinomatosis. Scale bars, 40 μm. ( g ) Immunohistochemical staining of β-catenin showing its nuclear delocalization in cancer cells and its overexpression at the tumour front. Scale bars, 40 μm. Full size image Remarkably, 38% of double-mutant NICD/p53 −/− mice developed tumours 5 months post induction, which were diagnosed as adenoma (42%) or adenocarcinoma (58%). All mice developed adenocarcinomas 15 months post induction ( Fig. 2b ). Compared with the single mutants, NICD/p53 −/− mice show a drastic increase in adenocarcinoma-related death ( Fig. 2a ), with an average of five tumours per animal. The tumours were predominantly located in the jejunum, ileum and rarely in the colon, and had a cystic appearance with irregular surfaces, and infiltrated the adjacent mesentery and fat tissue ( Fig. 2c ). Pathologically, tumours were classified as moderately or poorly differentiated (59.3% of total tumours) with complete invasion of the intestinal wall ( Fig. 2d ) characterized by muscularis and adipocyte infiltration. In addition, 56.7% of the most aggressive carcinomas had a moderate or severe desmoplastic stroma containing small groups of invading epithelial cells called budding cells ( Supplementary Table 1 ). Analysis of 30 compound mutant mice showed that 23.3% presented lymph node infiltration and 10% had liver metastases proving the capacity to disseminate in NICD/p53 −/− tumours. Fifty percent of the animals developed peritoneal carcinomatosis, with cancer cells infiltrating several tissues, including liver, spleen, diaphragm, mesentery and the abdominal wall. The histological characteristics of the 67 examined metastases revealed patterns resembling the primary tumours, including poor differentiation and moderate reactive stroma ( Fig. 2e and Supplementary Table 1 ). The intestinal origin of the cancer cells from the primary and secondary organs was confirmed by their GFP expression ( Fig. 2f ). Importantly, liver and lymph node metastases and peritoneal carcinomatosis are common implantation environments for metastases in patients with advanced CRC, demonstrating that the NICD/p53 −/− mutant mice efficiently mimic the metastatic spreading of the human disease. The Wnt pathway is known as the « gatekeeper » in the sequence of CRC mutation in human [36] . As readout of Wnt activation in our mouse model, we showed the occurrence of nuclear β-catenin mainly at the invasive front of the primary tumour and in secondary sites ( Fig. 2g ). The β-catenin target gene Fascin1 (ref. 37 ) was also overexpressed in the primary tumours and in metastases, but was absent in the normal epithelium ( Supplementary Fig. 3A ). In addition, other canonical Wnt target genes, c - Myc , Ccnd1 and Lgr5 were significantly overexpressed in total extracts of primary tumours compared with normal adjacent tissues ( Supplementary Fig. 3B–D ). Finally, by genome sequencing, we searched for mutations in four important Wnt factors ( Ctnnb1, Apc, Axin2 and Gsk3b ) comparing gene sequences in tumours versus normal tissue. In two of the eight individual NICD/p53 −/− pairs of samples, we detected 2 individual single-nucleotide variations in the exon 3 of the Ctnnb1 gene that correspond to the same frequency of hot spot mutations in the human CRC [38] . We also detected a stop gain mutation in the exon 16 of the Apc gene corresponding to a mutation described in human ( Supplementary Fig. 3E ). Taken together, these results showed that the Wnt pathway is activated in some NICD/p53 −/− primary tumours and their metastases. Concomitant activation of Notch and Wnt pathways triggers intestinal cell proliferation [29] that may provide an explanation for tumour initiation in this mouse model. However, regarding the numerous reports already published on digestive cancer initiation, we have not deciphered further the molecular mechanism responsible for the Wnt pathway activation, but specifically used our mouse model to study later steps of tumour progression and invasion [30] , [39] . EMT-like and invasion phenotype in NICD/p53 −/− tumours To test computationally derived hypothesis of synergistic NICD/p53 effect, we quantified the relative expression of 84 transcripts involved in EMT in tumours versus normal tissues. The majority of these genes were regulated as predicted, indicating activation of an EMT-like programme in the tumours ( P value=0.06; Supplementary Fig. 1A and Supplementary Table 2 ). We then compared the morphological and molecular features of the EMT-like process at the cellular level. In the desmoplasia of primary tumours, budding and single, potentially invasive cells were found ( Fig. 2d ). The observation of this cell type in the surrounding stroma suggests the existence of an EMT-like process. However, it is neither possible to discern the spatial boundaries of individual invasive cells nor determine their epithelial or mesenchymal origin by studying fixed, stained tissue. We therefore opted to study thick sections of live NICD/p53 −/− adenocarcinomas using two-photon microscopy and used GFP expression to track the fate of intestinal epithelial cancer cells in the tumours ( Fig. 3a ). While the majority of the primary tumours was GFP positive, we also observed numerous clusters and strings of GFP-positive epithelial cells further away from the primary tumour mass, lying in between thick collagen bundles, which suggested the presence of invading cancer cells ( Fig. 3b,c ). Importantly, we also illustrated the presence of isolated single GFP-positive cells exiting the tumour mass ( Fig. 3d ). 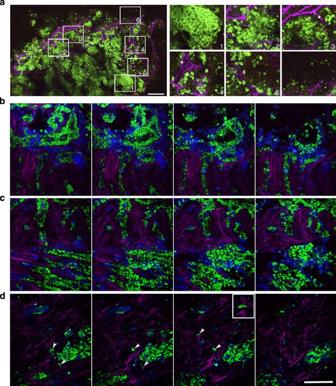Figure 3:Ex vivoanalysis of tumour slices by two-photon microscopy. (a)Ex vivotumour slice fromNICD/p53−/−mice observed by two-photon microscopy and represented as mosaic of 9 × 9 connected tiles. Epithelial cells have GFP-positive nuclei (green), second harmonic generation (SHG, pink) reveals the presence of collagen I. Insets represent higher magnification of several tumour areas (1–3 tumour bulk; 4–6 invasive areas). Scale bar, 100 μm. (b–d) Several examples ofex vivotumour slices fromNICD/p53−/−mice. Epithelial cells (GFP-positive nuclei, green), collagen I (SHG, pink), all cells (membrane dye, FM 4-64, blue). Images are taken from a Z-stack with 6 μm between planes. (b) Invasive front of the tumour. Note that stromal cells surround cancer cells. (c) Cancer cells invading stroma as clusters and strings parallel to the collagen fibres. (d) Cluster and single cancer cells invading collagen-rich stroma. Single cancer cells are labelled with white arrowheads. Inset, higher magnification of individual cancer cell with elongated nucleus. Scale bar, 100 μm. Figure 3: Ex vivo analysis of tumour slices by two-photon microscopy. ( a ) Ex vivo tumour slice from NICD/p53 −/− mice observed by two-photon microscopy and represented as mosaic of 9 × 9 connected tiles. Epithelial cells have GFP-positive nuclei (green), second harmonic generation (SHG, pink) reveals the presence of collagen I. Insets represent higher magnification of several tumour areas (1–3 tumour bulk; 4–6 invasive areas). Scale bar, 100 μm. ( b – d ) Several examples of ex vivo tumour slices from NICD/p53 −/− mice. Epithelial cells (GFP-positive nuclei, green), collagen I (SHG, pink), all cells (membrane dye, FM 4-64, blue). Images are taken from a Z-stack with 6 μm between planes. ( b ) Invasive front of the tumour. Note that stromal cells surround cancer cells. ( c ) Cancer cells invading stroma as clusters and strings parallel to the collagen fibres. ( d ) Cluster and single cancer cells invading collagen-rich stroma. Single cancer cells are labelled with white arrowheads. Inset, higher magnification of individual cancer cell with elongated nucleus. Scale bar, 100 μm. Full size image To further characterize the invading tumour cells from the primary tumour, we performed GFP lineage tracing in combination with the analysis of mesenchymal and epithelial markers by triple immunofluorescence staining ( Fig. 4a,e,i ). As expected, GFP-positive cells formed clusters ( Fig. 4b,f,j ), had an epithelial nuclear morphology and exclusively expressed epithelial markers such as ECAD ( Fig. 4b ), cytokeratin ( Fig. 4f ) and P120 ( Fig. 4j ). Interestingly, we observed that GFP-positive cells ( Fig. 4c,g,k ) detaching from the epithelial cluster lost their epithelial markers ECAD ( Fig. 4c ), Pan cytokeratin ( Fig. 4g ) and P120 ( Fig. 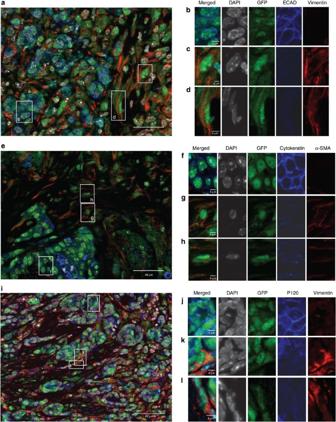Figure 4: An EMT-like phenotype is induced inNICD/p53−/−primary tumours. (a,e,i) Triple immunofluorescence of primary tumours using 4′,6-diamidino-2-phenylindole (grey) and GFP staining (green), an epithelial marker (blue) and a mesenchymal marker (red). Scale bars, 40 μm.b–d,f–h,j–lrepresent magnifications of the boxes lettered ina,e,i, respectively. (b,f,j) Clusters of epithelial cells express GFP and epithelial markers (ECAD, Pan cytokeratin and P120) but do not express mesenchymal markers (vimentin and α-SMA). (c,d,g,h,k,l) Single GFP-positive cells, with an epithelial origin, lose epithelial markers and acquire mesenchymal ones irrespective of whether they have epithelial (c,g,k) or fibroblast (d,h,l) nuclear morphology. Scale bars, 4 μm. 4k ), and acquired mesenchymal markers such as vimentin ( Fig 4c,k ) or α-SMA ( Fig. 4g ). Their nuclei, however, still had an epithelial-like morphology ( Fig. 4c,g,k ). At a later stage of morphological transition, we also observed GFP-positive cells with extended and elongated shapes exclusively expressing mesenchymal markers ( Fig. 4d,h,l ). Most of the GFP-positive cells in the desmoplastic area were still epithelial as they express ECAD (78%) or cytokeratin (81%), while ~20% of GFP-positive cells acquired a mesenchymal phenotype as indicated by vimentin or α-SMA expression. The acquisition of the mesenchymal phenotype characterized by vimentin or SMA expressing cells among GFP-positive cells highlights the significant negative correlation between vimentin and ECAD expressions (χ 2 test, P <0.0001) or between SMA and cytokeratin expressions (χ 2 test, P <0.0001) ( Fig. 5c ). The characteristic elongated shape of the nucleus was also observed in single GFP-positive cells in living tissue slices ( Fig. 3d , insert). Notably, we observed a strong nuclear β-catenin staining in cells exiting the primary tumour ( Fig. 2g ), thereby confirming our predictions that EMT inducers participate in the Wnt pathway activation. In addition, the mesenchymal marker N-cadherin was also acquired in tumour cells invading the desmoplastic area ( Fig. 5a ). Together, these results demonstrate the existence of epithelial GFP-positive cells that have undergone a complete EMT-like transition with a full mesenchymal phenotype. Figure 4: An EMT-like phenotype is induced in NICD/p53 −/− primary tumours. ( a , e , i ) Triple immunofluorescence of primary tumours using 4′,6-diamidino-2-phenylindole (grey) and GFP staining (green), an epithelial marker (blue) and a mesenchymal marker (red). Scale bars, 40 μm. b – d , f – h , j – l represent magnifications of the boxes lettered in a , e , i , respectively. ( b , f , j ) Clusters of epithelial cells express GFP and epithelial markers (ECAD, Pan cytokeratin and P120) but do not express mesenchymal markers (vimentin and α-SMA). ( c , d , g , h , k , l ) Single GFP-positive cells, with an epithelial origin, lose epithelial markers and acquire mesenchymal ones irrespective of whether they have epithelial ( c , g , k ) or fibroblast ( d , h , l ) nuclear morphology. Scale bars, 4 μm. 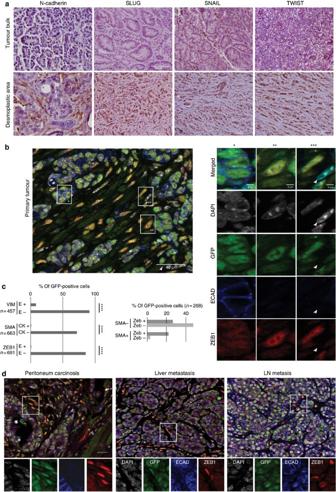Figure 5: Characterization of an EMT-like phenotype inNICD/p53−/−primary tumours. (a) Staining of the mesenchymal marker N-cadherin and the EMT transcription factors, SNAIL, SLUG and TWIST inNICD/p53−/−primary tumours. Left panel: N-cadherin is overexpressed in tumour cells invading the desmoplastic area compared with those from the tumour bulk. Scale bars, 40 μm. Middle and right panels: a nuclear overexpression of EMT transcription factors is observed in cancer cells from the desmoplastic area compared with differentiated tubular structures. Scale bars, 100 μm. (b,c) Expression of the EMT-inducer ZEB1 in primary tumours ofNICD/p53−/−. (b) Left panel: triple immunofluorescence onNICD/p53−/−primary tumours using 4,6-diamidino-2-phenylindole (DAPI; grey) and GFP staining (green), ECAD (blue) and ZEB1 (red). Scale bars, 40 μm. Right panel: magnification of different tumour cell features coming from the same slide showing that cells undergoing EMT-like processes express the EMT-inducer ZEB1. *Zeb1 negative epithelial tumour cells; ** and *** Zeb1 and GFP-positive, ECAD-negative cells, independently of their morphology. Scale bars, 4 μm. The white arrow labels individual ZEB1-negative cells with a non-epithelial origin. (c) The left bar graph shows the frequency of vimentin, SMA or Zeb1-positive cells among GFP-positive cells. Cells were separated in two groups presenting either an epithelial phenotype described by ECAD-positive cells (E+) or cytokeratin-positive cells (CK+), or an EMT-like phenotype characterized by ECAD negative (E−) or CK negative (CK−). The associated tables of contingency (Supplementary Table 4) depict a strong negative correlation (***) between ZEB1 and ECAD expressions (P<0.001), vimentin and ECAD expressions (χ2test,P<0.001) or SMA and CK expressions (χ2test,P<0.001). The right bar graph shows the distribution of Zeb1 and SMA among GFP positive cells. ZEB1 is expressed in SMA-negative cells in 27% of GFP-positive cells and in SMA-positive cells for 22.4% GFP-positive cells. Only 3% of GFP-positive are ZEB1-negative cells and SMA positive, suggesting that a small fraction of cells have fully completed the EMT process. (d) Triple immunofluorescence onNICD/p53−/−metastatic tissues using DAPI (grey), GFP staining (green), ECAD (blue) and ZEB1 (red; scale bars, 20 μm) with magnifications of one area showing the presence of GFP-intestinal cancer cells with mesenchymal features in the secondary organs (scale bars, 4 μm). Full size image Figure 5: Characterization of an EMT-like phenotype in NICD/p53 −/− primary tumours. ( a ) Staining of the mesenchymal marker N-cadherin and the EMT transcription factors, SNAIL, SLUG and TWIST in NICD/p53 −/− primary tumours. Left panel: N-cadherin is overexpressed in tumour cells invading the desmoplastic area compared with those from the tumour bulk. Scale bars, 40 μm. Middle and right panels: a nuclear overexpression of EMT transcription factors is observed in cancer cells from the desmoplastic area compared with differentiated tubular structures. Scale bars, 100 μm. ( b , c ) Expression of the EMT-inducer ZEB1 in primary tumours of NICD/p53 −/− . ( b ) Left panel: triple immunofluorescence on NICD/p53 −/− primary tumours using 4,6-diamidino-2-phenylindole (DAPI; grey) and GFP staining (green), ECAD (blue) and ZEB1 (red). Scale bars, 40 μm. Right panel: magnification of different tumour cell features coming from the same slide showing that cells undergoing EMT-like processes express the EMT-inducer ZEB1. *Zeb1 negative epithelial tumour cells; ** and *** Zeb1 and GFP-positive, ECAD-negative cells, independently of their morphology. Scale bars, 4 μm. The white arrow labels individual ZEB1-negative cells with a non-epithelial origin. ( c ) The left bar graph shows the frequency of vimentin, SMA or Zeb1-positive cells among GFP-positive cells. Cells were separated in two groups presenting either an epithelial phenotype described by ECAD-positive cells (E+) or cytokeratin-positive cells (CK+), or an EMT-like phenotype characterized by ECAD negative (E−) or CK negative (CK−). The associated tables of contingency ( Supplementary Table 4 ) depict a strong negative correlation (***) between ZEB1 and ECAD expressions ( P <0.001), vimentin and ECAD expressions (χ 2 test, P <0.001) or SMA and CK expressions (χ 2 test, P <0.001). The right bar graph shows the distribution of Zeb1 and SMA among GFP positive cells. ZEB1 is expressed in SMA-negative cells in 27% of GFP-positive cells and in SMA-positive cells for 22.4% GFP-positive cells. Only 3% of GFP-positive are ZEB1-negative cells and SMA positive, suggesting that a small fraction of cells have fully completed the EMT process. ( d ) Triple immunofluorescence on NICD/p53 −/− metastatic tissues using DAPI (grey), GFP staining (green), ECAD (blue) and ZEB1 (red; scale bars, 20 μm) with magnifications of one area showing the presence of GFP-intestinal cancer cells with mesenchymal features in the secondary organs (scale bars, 4 μm). Full size image To further characterize the changes that are responsible for an EMT-like process in NICD/p53 −/− tumour cells, we analysed the expression of the EMT inducers, Slug, Snail, Twist and Zeb1 (refs 40 , 41 , 42 , 43 , 44 ). The four of the EMT inducers were upregulated in the primary tumours compared with normal tissue ( Supplementary Table 2 ). Immunohistochemistry showed that while SLUG, SNAIL and TWIST were not expressed in the nuclei of cells present in the non-invasive area, they were expressed specifically in nuclei of cells in the invading desmoplastic area in which EMT-like cells were found ( Fig. 5a ). For ZEB1 expression, we were able to use the triple immunostaining approach ( Fig. 5b ) to show that although ZEB1 was not expressed in epithelial tumour cells (indicated by * in Fig. 5b ), it was induced in isolated GFP-positive, ECAD-negative cells, independently of their morphology (indicated by ** and *** in Fig. 5b ). Notably, GFP-negative cells with mesenchymal phenotypes are not necessary marked by ZEB1 (indicated by *** in Fig. 5b labelled with arrow). Interestingly, quantification of ZEB1- and ECAD-positive and -negative cells among GFP-positive cells highlights the significant negative correlation between ZEB1 and ECAD expressions ( P <0.0001) ( Fig. 5c , left panel). Analysis of ZEB1 and α-SMA among the GFP-positive cells indicate that half of the ZEB1-positive cells are also α-SMA positive, whereas only a small fraction of α-SMA-positive cells are ZEB1 negative, thereby suggesting a fully completed EMT process ( Fig. 5c , right panel). For further analysis of the dynamics of EMT-like cells, we evaluated the expressions of ZEB1 and ECAD in the invaded lymph node, liver and peritoneal carcinomatosis ( Fig. 5d ). While the vast majority of metastatic cancer cells have an epithelial feature by expressing ECAD but not ZEB1, cells with an EMT-like phenotype also existed. The presence of ZEB1-positive ECAD-negative cells arising from intestinal epithelial tumours confirmed previous work on the conserved cell plasticity of EMT-like cells in the three secondary sites [12] . However, the fact whether these cells are fuelling the tumour or about to leave it, remains unanswered. According to network analysis, the shift to an EMT-like phenotype in NICD/p53 −/− mutants is associated with a decreased cell proliferation via regulation of transcription and subcellular localization of p21, which is in agreement with studies in tumour cell lines [45] . We validated this prediction in the NICD/p53 −/− mice by demonstrating nuclear localization of p21 ( Fig. 6a ) and a reduction in mitotic cells ( Fig. 6b–e ) among EMT-like cells found in the desmoplastic region of the tumour. Indeed, while 12% of the GFP-positive epithelial cells are proliferative, only 2% of EMT-like cells are mitotic (χ 2 test, P <0.01; Fig. 6f ). 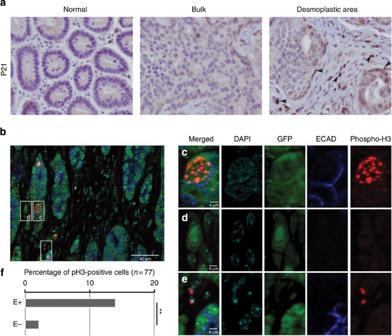Figure 6: EMT-like cells are not proliferative. (a) Immunohistochemical staining of P21 inNICD/p53−/−primary tumours, showing nuclear P21 expression in cancer cells at the tumour front. This feature is emphasized in cancer cells invading the desmoplastic area. Scale bars, 100 μm. (b) Triple immunofluorescence onNICD/p53−/−primary tumours using 4′,6-diamidino-2-phenylindole (grey), GFP staining (green), ECAD (blue) and phospho-H3 (red). Scale bars, 40 μm. (c–e) Magnification of different tumour cell features coming from the same slide showing some epithelial cells in clusters (c) or fibroblasts (e) in division whether EMT-like cells are quiescent (d). Scale bars, 4 μm. (f) Proportion of pH3-positive cells among GFP-positive cells. Among GFP-positive cells, 12% of cells with an epithelial morphology as defined by ECAD positivity (E+;n=585) are proliferative, while only 2% of ECAD-negative cells (E−;n=274) express pH3 (full contingency table indicates dependency χ2test,P<0.0001, **). This indicates that cells undergoing EMT-like are less proliferative. Figure 6: EMT-like cells are not proliferative. ( a ) Immunohistochemical staining of P21 in NICD/p53 −/− primary tumours, showing nuclear P21 expression in cancer cells at the tumour front. This feature is emphasized in cancer cells invading the desmoplastic area. Scale bars, 100 μm. ( b ) Triple immunofluorescence on NICD/p53 −/− primary tumours using 4′,6-diamidino-2-phenylindole (grey), GFP staining (green), ECAD (blue) and phospho-H3 (red). Scale bars, 40 μm. ( c – e ) Magnification of different tumour cell features coming from the same slide showing some epithelial cells in clusters (c) or fibroblasts (e) in division whether EMT-like cells are quiescent (d). Scale bars, 4 μm. ( f ) Proportion of pH3-positive cells among GFP-positive cells. Among GFP-positive cells, 12% of cells with an epithelial morphology as defined by ECAD positivity (E+; n =585) are proliferative, while only 2% of ECAD-negative cells (E−; n =274) express pH3 (full contingency table indicates dependency χ 2 test, P <0.0001, **). This indicates that cells undergoing EMT-like are less proliferative. Full size image In summary, in agreement with computational predictions, we demonstrate a global activation of the EMT-like programme in NICD/p53 −/− primary tumours and metastases. These results emphasized the existence of EMT in cancer and its importance in cancer progression. Human data analysis To confirm the relevance of our study for human disease, we analysed the presence of EMT-like cells in primary CRC and liver metastasis from human patients. The importance of ZEB1 in cancer progression, in particular, in promoting cancer invasion and metastasis has already been described [4] , [42] , [44] , [45] . Moreover, this EMT inducer is overexpressed in human CRC and more specifically in dedifferentiated tumour cells in the tumour front [46] . Our model confirmed that ZEB1 could be used as a marker for EMT process ( Fig. 5b ). We thus used this marker together with ECAD expression to study the EMT-like process in invading human cells from the primary tissue to the secondary organs. Although ZEB1 is not expressed in the bulk of the primary tumour, invading cells are strongly stained for ZEB1 ( Fig. 7a,b ). Similarly, ZEB1-positive/ECAD-negative cells are present in liver metastases, either close to an epithelial cluster or surrounded by liver cells ( Fig. 7c–f ). These observations suggest that an EMT-like process also occurs in human invasive adenocarcinomas and in their metastases. 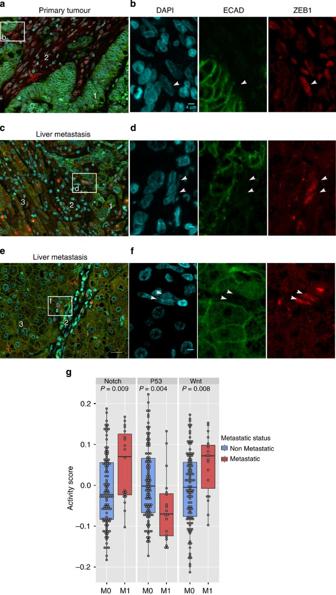Figure 7: EMT signalling activation in human samples with CRC. (a–f) Double immunofluorescence on human samples with CRC using ZEB1 (red) and ECAD (green). (a) CRC primary tumour and (c,e) liver metastasis, showing ZEB1-positive/ECAD-negative cells invading the desmoplastic area in primary tumour and in liver metastasis. Numbers ona,c,eindicate different cell types observed on the slide as follows: 1 for colorectal primary (ina) or metastatic cells (inc), 2 for stroma cells and 3 for hepatocytes. Scale bars, 20 μm. Magnifications from the boxes b,d,f are also represented inb,d,fsingle 4′,6-diamidino-2-phenylindole, ECAD and ZEB1 staining. ZEB1-positive cells (labelled with an arrowhead) in the liver metastasis are either observed next to colorectal tumour cells (d) or surrounded by hepatic tissue (f). Scale bars, 4 μm. (g) The activity scores computed for the Notch, p53 and Wnt pathways in human colon cancer samples from Tumour Cancer Genome Atlas data set. The data points represent primary tumour samples grouped as non-metastatic (blue) and metastatic (red) according to the observation of distant metastases. The bottom and top of the box correspond to the first and third quartiles of the activity score values, and the band inside the box represents the median.Pvalues are calculated using the two-samplet-test between the two groups. Figure 7: EMT signalling activation in human samples with CRC. ( a – f ) Double immunofluorescence on human samples with CRC using ZEB1 (red) and ECAD (green). ( a ) CRC primary tumour and ( c , e ) liver metastasis, showing ZEB1-positive/ECAD-negative cells invading the desmoplastic area in primary tumour and in liver metastasis. Numbers on a , c , e indicate different cell types observed on the slide as follows: 1 for colorectal primary (in a ) or metastatic cells (in c ), 2 for stroma cells and 3 for hepatocytes. Scale bars, 20 μm. Magnifications from the boxes b,d,f are also represented in b , d , f single 4′,6-diamidino-2-phenylindole, ECAD and ZEB1 staining. ZEB1-positive cells (labelled with an arrowhead) in the liver metastasis are either observed next to colorectal tumour cells ( d ) or surrounded by hepatic tissue ( f ). Scale bars, 4 μm. ( g ) The activity scores computed for the Notch, p53 and Wnt pathways in human colon cancer samples from Tumour Cancer Genome Atlas data set. The data points represent primary tumour samples grouped as non-metastatic (blue) and metastatic (red) according to the observation of distant metastases. The bottom and top of the box correspond to the first and third quartiles of the activity score values, and the band inside the box represents the median. P values are calculated using the two-sample t -test between the two groups. Full size image To further verify in human the importance of Wnt, p53 and Notch pathways in EMT induction, we used a publicly available human colon cancer gene expression data set and compared the activity scores of Notch, Wnt and p53 pathways in cancer progression. We revealed that Notch and Wnt pathways were significantly activated, whereas the p53 pathway was downregulated in the metastatic compared with non-metastatic tumours ( Fig. 7g ). Moreover, concerning Notch target genes expression, nuclear staining for NICD and Hes1 in few cells invading the stroma of human invasive colon adenocarcinoma illustrate the activation of Notch signalling at the invasive front of human CRC ( Supplementary Fig. 4B ). These results collectively confirm the major role of these pathways in metastasis development and correlate with our mouse model to suggest a possible mechanism leading to EMT induction through the Notch pathway activation in the context of p53 reduction. In this study, we aimed to create a mouse model of EMT-like induction in intestinal cancer followed by metastasis. Here we show that the computational analysis of a comprehensive signalling network suggest the crosstalk between Notch, p53 and Wnt pathways as a possible determinant of EMT induction. In agreement with our analysis, no EMT-like phenotype was observed in Apc −/− (ref. 30 ), NICD [28] and NICD/Apc −/− (ref. 29 ) transgenic mouse models. Also coherent with our p53 −/− predictive model, EMT has been shown to be inhibited by p53 in the Braf V637E mice [27] . On the contrary, our hypothesis based on the signalling network analysis about the synergy between NICD induction and p53 loss to trigger EMT has been confirmed by the NICD/p53 −/− mice using GFP lineage tracing, even if the use of a p53-mutated model would have been more relevant with the human disease [27] . Finally, to demonstrate the relevance of the new transgenic mice to human disease, we show that in the invasive human colon cancer samples and their related metastases, EMT markers were enhanced together with a negative regulation of epithelial markers. This phenotype in human samples is associated with modulation of Notch , Wnt and p53 gene expression in similar manner as in the mice model, supporting a synergy between these genes to permit EMT induction. Our prediction of synthetic interaction between Notch and p53, which we confirmed experimentally, demonstrated that there are additional ways to reach permissive conditions that induce EMT in addition to those already described in the literature. Although we have not investigated in detail how the Wnt pathway was implicated in the NICD/p53 −/− mice, we have observed two independent single-nucleotide variations on the Ctnnb1 gene corresponding to hot spot mutations in human CRC [38] and a stabilization of β-catenin [24] , resulting in a hyperactivation of Wnt signalling at the invasive front of the tumour, in EMT-like cells and in metastasis. This result is concordant with a recent work showing that upon loss of cell-to-cell contact, phosphorylation of β-catenin reduced its association with ECAD and expanded signalling responsible for EMT induction [47] . How the Wnt pathway is precisely activated in NICD/p53 −/− tumours was not directly investigated, although based on the network analysis we hypothesize that the Wnt pathway is regulated by Notch during the induction of EMT programme. While some papers indicate a negative regulation of β-catenin by Notch [48] , other works suggest an activation of the Wnt signalling through Notch-dependent EMT inducers [24] . The Wnt pathway, in turn, can induce the expression of Notch pathway factors, in this way creating a positive feedback loop [25] . We have previously reported the effects associated with Notch activation on the onset of colorectal tumour development [29] . In this study, we have extended our previous observations and shown a crucial role for Notch signals during later stages of cancer progression as illustrated by Hes1 staining in NICD/p53 −/− tumours ( Supplementary Fig. 4A ). While Notch signalling is downregulated in the bulk of adenocarcinomas compared with adenomas, the importance of this signalling pathway in the latter stage of tumour development has already been proposed by the Taketo’s group [49] . However, further characterization may be required to determine whether Aes affects CRCs through Notch or other signalling pathways. Notch activation could be achieved through several distinct mechanisms, such as epigenetic control of positive or negative regulators of the Notch pathway, eventually leading to more active Notch signalling. Regarding its regulation, it has recently been shown in colon cancer stem cells that a complex Notch regulation by mir34 or Numb was implicated in cell fate decision [50] . Despite this microRNA-regulated mechanism, how Notch signalling is modulated during tumour progression and in invasion specifically in colon is still under investigation. Notch has been shown in many cancers to have a role as a direct regulator of major EMT transcription factors SNAIL, SLUG, TWIST, ZEB1, and ZEB2 (refs 19 , 40 , 51 ) that consequently triggers an EMT-like programme. In turn, SNAIL and TWIST stabilize β-catenin [24] . Important components of Wnt and Notch pathways are negatively regulated by miRNAs induced by members of the p53 family (p53, p63 and p73) [52] . Thus, the balance between positive (Notch and Wnt) and negative (p53, p63, p73 and miRNAs) regulatory circuits on EMT inducers will dictate the resulting phenotype. Our transgenic mouse model represents an excellent model for understanding the balance of the Notch, Wnt and p53 molecular mechanisms and other signalling pathways to induce EMT in colon cancer. The role of microenvironment in conditioning cancer cell to undergo EMT-like process should be taken into account. Understanding whether paracrine signals from the stroma and immune-competent cells are involved in EMT-like will be essential for determining how to control and target EMT-like cells to impair tumour dissemination. Indeed, in the NICD/p53 −/− mice, Notch and p53 are altered in every carcinoma cells, but only a small portion of these cells will undergo an EMT-like transition, which is in accordance with other observations [12] ( Fig. 8 ). EMT-like phenotype is not only a consequence of genetic mutations appearing in cancer cells. Indeed, the role of endogenous signals for the induction of EMT, such as transforming growth factor-β, the extracellular matrix and inflammatory signals from the surrounding stroma, also contribute in the conversion of EMT phenotype necessary for tumour invasion and migration [53] , [54] . Moreover, it has been reported that Notch signals can be activated in CRC cells by endothelial cells in a paracrine manner [49] , [55] . This could explain why Notch signals are specifically activated at the tumour front. Thus, the NICD/p53 −/− mice model provides also an opportunity to study the role of the microenvironment in development of metastases, thanks to the lineage tracer technology. Following the evolution of cancer cells from non-invasive to invasive and then metastatic and in parallel, dissecting the composition of stroma and ECM surrounding the cancer cell will help shading light on the role of extracellular signals on EMT-like process. 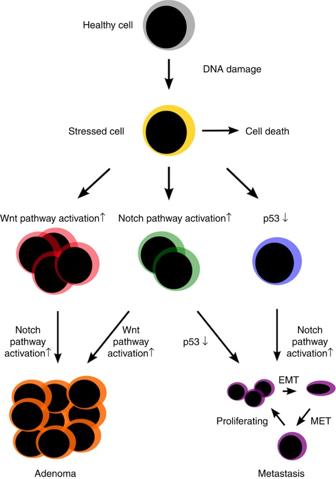Figure 8: Schematic representation of phenotypes observed in single and double mutants. When DNA damage occurs in a healthy cell, the cell can undergo apoptosis if the damage is severe enough. If another mutation then occurs, this can lead to different cell phenotypes depending on the kind of mutation:Apcloss-of-function mutation, as well asNotchactivation will give rise to increased proliferation. Ap53loss-of-function mutation will give rise to a cell phenotype that is able to survive, as apoptosis can no longer be induced by p53. A sequential mutation will lead to either adenoma or metastases depending on the preceding mutation. MET: mesenchymal epithelial transition. The predicted phenotypes have been confirmed by experiments. Figure 8: Schematic representation of phenotypes observed in single and double mutants. When DNA damage occurs in a healthy cell, the cell can undergo apoptosis if the damage is severe enough. If another mutation then occurs, this can lead to different cell phenotypes depending on the kind of mutation: Apc loss-of-function mutation, as well as Notch activation will give rise to increased proliferation. A p53 loss-of-function mutation will give rise to a cell phenotype that is able to survive, as apoptosis can no longer be induced by p53. A sequential mutation will lead to either adenoma or metastases depending on the preceding mutation. MET: mesenchymal epithelial transition. The predicted phenotypes have been confirmed by experiments. Full size image The ability of cancer cells to metastasize from the primary organ to secondary sites involves their capacity to invade adjacent tissue. However, while collective invasion of tumour cells is commonly admitted, single migration of cancer cells is difficult to demonstrate using morphologic criteria and standard markers. Here, by lineage tracing of the cancer cells in a transgenic mouse model, we have confirmed in the digestive tract what has been previously observed in pancreatic cancer by demonstrating in vivo the occurrence of an EMT-like process associated with metastatic disease progression [14] . From the initial loss of epithelial markers to the complete acquisition of mesenchymal phenotype, EMT-like cells undergo a complete reorganization. Previous descriptions of malignant cells with combined expression of epithelial and mesenchymal markers in vivo in mouse models and in human tumours have suggested the presence of partial EMT-like in cancer [56] . Indeed, cancer cells co-expressing both cytokeratins and vimentin have been identified in breast cancers [57] . In our study, expression of epithelial origin tracker in mesenchymal cells emphasizes the plasticity of these cells that are able to initiate and reach completion of their EMT-like process ( Supplementary Table 3 ). While our mouse model allows clear analysis of EMT-like cells with epithelial origin, it does not provide tracing of single EMT-like cell to follow contribution of its progeny in dissemination and metastasis. The concept of an EMT-like phenotype is frequently associated with the reverse process called mesenchymal-to-epithelial transition (MET) owing to the similarities between primary tumours and metastases at the histologic level. Interestingly, in this study, we visualize the presence of cancer cells with mesenchymal features in the secondary site, reinforcing the plasticity of EMT-like cells in the secondary organs. However, we cannot conclude from our observation whether these cells are arriving or leaving the secondary site where epithelial GFP cells are also found. Despite the progress in intravital imaging approaches to provide quantitative and dynamic insight in living animals [58] , its use to follow EMT-like migration on the whole body remains very challenging. In clinic, the presence of cells with some EMT properties is strongly associated with metastatic progression [59] . The master regulators of embryonic EMT programmes are frequently aberrantly expressed in various types of carcinomas and associated with bad prognosis. The development of high-grade invasive adenocarcinomas that give rise to liver metastasis and peritoneal carcinomatosis with tracer of cancer cells in NICD/p53 −/− mice makes them a relevant mouse model for aggressive human CRC and a good system for therapeutic drugs discovery in invasive cancer. By combining intravital imaging progresses, colonoscopy engineering and the role of EMT-like cells in cancer progression, cancer therapy targeting EMT-like tumour cells could be conveniently tested in our mouse model. Ethics statement All mice were kept in the Curie Institute-specified pathogen-free animal area for mouse breeding and experimental purpose (facility licence no, B75-05-18) under the authority of the Institute’s veterinarian Virginie Dangles-Marie. The care and use of animals used in this facility is strictly applying to European and national regulation for the protection of vertebrate animals used for experimental and other scientific purposes (Directive 86/609 and 2010/63). Transgenic mouse models All mice used in this work have been previously described: villin-CreERT2 mice [32] , p53 mice (referred as p53 −/− ) [26] and the Rosa-N1ic mice (referred as NICD ) [33] . These strains crossed for >10 generations to reach an isogenic C57BL/6 background that have been used to generate the p53 −/− , NICD and NICD/p53 −/− compound mice. Genotyping of littermates was performed using the primers listed in Supplementary Information . Special care was taken to eliminate compound mice with a double copy of the villin-CreERT2 transgene. Four-week-old mice, including all control mice, were injected intraperitoneally with tamoxifen (50 μg kg −1 of animal body weight) for 5 consecutive days. Every 2 months, at least five littermates from each compound mouse line were killed and macroscopically analysed to evaluate tumour development. Survival probabilities were estimated by Kaplan–Meier analysis, according to ethical committee guidelines, considering the presence or absence of adenocarcinoma as an event at the death of the animal. Deep macroscopic and microscopic analyses were performed on tumours and metastases from these animals. Genotyping of littermates was performed using the following primers: for Notch, N5: 5′-AAAGTCGCTCTGAGTTGTTAT-3′, N3: 5′-GAAAGACCGCGAAGAGTTTG-3′ and Rosa: 5′-TAAGCCTGCCCAGAAGACTC-3′. N5 and Rosa or N5 and N3 primers detect presence of WT or NICD, respectively. The presence of the Cre recombinase is detected using Cre (F): 5′-CAAGCCTGGCTCGACGGCC-3′ and Cre (R): 5′-CGCGAACATCTTCAGGTTCT-3′. The use of P53 (F): 5′-CACAAAAACAGGTTAAACCCAG-3′ and P53 (R): 5′-AGCACATAGGAGGCAGAGAC-3′ primers allows amplification of a 288-pb fragment in case of WT P53 or a 370-pb fragment when P53 is floxed. Construction of the signalling network The signalling network map of EMT regulation was manually constructed and based on curated information extracted from the literature retrieved from the PubMed database. The map is assembled using the CellDesigner tool [60] and the Systems Biology Graphical Notation [61] standard for representing molecular biology mechanisms. The software creates a structured network representation in Systems Biology Markup Language, suitable for further computational analysis [62] . Corresponding references and specific notes annotate each entity of the map. Literature selection rules The rules for literature selection are the following: first 5–10 review articles in the field were chosen for extracting the consensus pathways and regulations accepted in the field and for approaching to the literature suggested in these review. This allowed us to construct the ‘backbone’ of the network map and to define the boundaries of pathways coverage. Further, information from original papers, preferably most recent studies, is analysed and added to enlarge and enrich the map. The decision about adding a biochemical mechanism to the map has to be supported by at least two independent studies performed in different teams. Further, the coherence of the signalling network map has been verified by checking that they predict observed phenotypes of single and double mutants that have already been described in experimental models. Our map of the signalling network of EMT regulation is based on information extracted from 135 scientific papers ( http://navicell.curie.fr/pages/signalling_network_emt_regulation_description.html ). Signalling network map content The signalling network map contains about 400 chemical species representing proteins and their modifications, molecular complexes, RNAs, miRNAs, genes, phenotypes and regulatory influences formed by ~400 biochemical reactions. The map contains regulatory circuits connected to phenotypes such as proliferation, apoptosis and EMT, and others. The content of the map has been validated by comparison with the map derived from the Ingenuity database using as inputs Notch, p53, Wnt, apoptosis, EMT and proliferation. The Notch–p53–Wnt signalling network can be explored interactively at http://navicell.curie.fr/pages/signalling_network_emt_regulation_description.html , using NaviCell, an online tool for navigating large signalling maps [63] . Structural analysis of signalling network Analysis of the map was performed using the BiNoM plugin in Cytoscape [64] . Path analysis and node neighbourhood study were carried out for extracting major signalling paths that affect EMT, proliferation and apoptosis phenotypes, and for conversion of the signalling network model into an influence diagram. We performed a complexity reduction of the influence diagram in four steps, each decreasing the level of details to produce reduced network models ( Supplementary Fig. 2 ). This reduction allowed us to eliminate those factors on the map that did not affect studied phenotypes, to understand organization principles of the map and to find core paths on the network preserved through all reduction levels. In this way, the regulatory patterns recapitulating the signalling mechanisms regulating three phenotypes were identified, and single and double mutants were analysed using the reduced models. Reduced models of level 3 and 4 were used for illustrating molecular phenotypes in WT and mutant cells. Histology and immunohistochemistry staining and analysis Freshly dissected intestinal tumours and metastases were either fixed in 4% neutral-buffered paraformaldehyde for 2 h and paraffin embedded, or snap-frozen in cooled isopentane. Paraffin sections (4 μm) were either haematoxylin and eosin stained for histological analysis or subjected to immunostaining. An experienced veterinary pathologist performed histological analyses on tissues from 30 NICD/p53 −/− mice (103 primary tumours and 67 metastases). For staining, paraffin-embedded samples were deparaffinized and rehydrated before being subjected to antigen retrieval with 10 mM boiling sodium citrate, pH 6, for 20 min. For immunohistochemistry, endogenous peroxidase were then blocked by a 1.5% H 2 O 2 in PBS treatment for 20 min. Slides were then incubated for 1 h with a nonspecific binding blocking solution (5% normal bovine serum in PBS) followed by the corresponding primary antibody, overnight at 4 °C. For immunohistochemistry, samples were incubated with biotinylated-conjugated secondary antibodies for 45 min followed by incubation with ABC for 30 min (Elite) and visualized using DAB peroxidase substrate kit (Vector Labs). Slides were then counterstained with haematoxylin and mounted in polymount xylene (Polysciences). For immunofluorescence, slides were incubated with fluorochrome-conjugated secondary antibody and 4′,6-diamidino-2-phenylindole for 1 h and mounted in Vectashield medium (Vector Labs). Representative images from immunofluorescence and immunohistochemistry stainings were acquired using an Apotome system with a × 40 water Plan-Apochromat lens (Zeiss, Jena, Germany) or an epifluorescence microscope (Nikon, C-HGFIE), respectively. All images were further processed and pseudo-coloured using ImageJ (National Institutes of Health). A special staining protocol was performed for β-catenin staining, as previously described. Briefly, Tris-EDTA, pH 9, solution was used for antigen retrieval and peroxidase blocking was achieved in buffer containing 15 mM NaN 3 , 50 mM Na 2 HPO 4 , 20 mM citric acid and 1.5% H 2 O 2 . Antibody references and working dilution were used as follow: ECAD (BD-610182, 1/400), vimentin (CS-5741, 1/300), GFP (ab 13970, 1/300), Pan cytokeratin (Dako ZO622, 1/200), α-SMA (Sigma A2547, 1/600), SLUG (CS-9585, 1/100), SNAIL (ab 85931, 1/100), TWIST (sc-15393, 1/100), ZEB1 (Euromedex 00419, 1/200), β-catenin (BD-610154, 1/50), FASCIN1 (Dako M3567, 1/50), P21 (ab 2961, 1/150), phospho-H3 (Millipore 06570, 1/1000), NICD (sc-6014, 1/100) and HES1 (Clinisciences D134-3, 1/50), P120 (BD-610133, 1/100), P53 (Dako DO-7, 1/200) and N-cadherin (Zymed 3B9, 1/100). Image analysis To quantify the triple immunofluorescence images presented in Figs 5 and 6 , cells were counted in defined categories on the maximum intensity projection of immunofluorescence image stacks, defining 2 × 2 contingency tables ( Supplementary Table 4 ). A total of 5–9 acquisitions were processed for each combination of immunofluorescence antibodies. Test of significance of contingency tables were performed using the Prism software with a χ 2 -analysis. Statistical analysis Statistical analyses were performed with the Prism software. This leads to the quantification of the number of cells as a contingency table associated with a χ 2 -analysis. Two-photon imaging A piece of intestine containing a tumour was isolated from an 8-month-old tamoxifen-injected NICD/p53 −/− mouse. The intestinal explant was flushed with PBS containing 1% penicillin/streptomycin and 0.5% gentamycin. For some experiments, explants were incubated for 15 min at room temperature in 40 μg ml −1 FM 4-64 FX dye (Invitrogen). The explant was filled with and embedded in 4% (wt/vol) low-melting agarose (Invitrogen) pre-warmed at 37 °C. A vibratome (Leica VT1000S) was used to slice the tumour into 500 μm sections with a velocity of 0.125 mm s −1 and a vibration frequency of 70 Hz. The tissue was transferred to a 35-mm tissue culture dish containing 2 ml of culture medium DMEM-Glutamax (Gibco) supplemented with 1% penicillin/streptomycin, 2.5% fetal bovine serum, 0.25 U ml −1 insulin (Sigma-Aldrich), 100 μg ml −1 transferrin (Holo, Human Plasma, Calbiochem) and 10 ng ml −1 murine epidermal growth factor (Peprotech). Tissue explant was maintained at 37 °C and imaged using two-photon laser-scanning microscopy using a LSM510 Meta (Zeiss) coupled to a MaiTaiDeepSee femtosecond laser (690–1,020 nm; Spectra-Physics, Mountain View, CA, USA), using an Zeiss Achroplan × 40/NA (numerical aperture) 1.0 water immersion objective. Fluorescence channels were recorded simultaneously with a 555-nm dichroic mirror in combination with 472/30 (second harmonic generation), 520/35 (GFP) and 585/40 (Tomato) band-pass filters. The excitation wavelength was 920 nm. Three-dimensional stacks were obtained for up to 250 μm penetration depth at a step size of 3 μm. Standard contrast and intensity levels were further adjusted using Photoshop CS5 (Adobe). Exome sequencing of four genes of the Wnt pathway Genomic DNA was isolated from paraffin-embedded tissue of eight different mice. Each intestinal tumour sample was sequenced using the Ion Torrent PGM technology and matched with a control sample from liver or node. A dedicated sequencing panel targeting the coding part of the genes Ctnnb1, Gsk3b, Axin2 and Apc was used. Sequenced reads were then aligned of the mm10 reference genome using the TMAP software (v 3.6.3-1, Life Technologies). Around 80% of the reads were aligned on the targeted genes with a mean depth of coverage of × 1,500. The calling of somatic variants was performed using the pair of tumour and control samples using the Varscan software (v. 2.3.6; ref. 65 ). Finally, the list of variants was annotated using the ANNOVAR software [66] in order to facilitate their functional interpretation. Human samples Sixteen invasive adenocarcinomas were obtained from the Gastroenterology and Pathology Unit of the Curie Institute in Paris, with written consent of the patients and approval of the local ethics committee. Patients included in this study had developed synchronous or metachronous liver metastasis. Quantification of pathway activities in human tumours We used the publicly available colon cancer gene expression data set from Tumour Cancer Genome Atlas [67] to compare the activities of Notch, Wnt and p53 pathways in metastatic and non-metastatic human colon tumour samples. Excluding rectum cancers from the original data set, we left with 121 colon cancer samples included in our analysis. Since single gene-based analysis did not show significant differential changes in gene expression of Wnt, β-catenin, Notch and p53 genes (data not shown), we analysed the expression of their downstream targets recapitulated into a pathway activity score. The pathway activity score in a tumour sample was defined as contribution of this sample into the first principal component computed for all samples on the set of the pathway target genes, as it was done in ref. 68 . Molecular Signature Database [69] was used to select the sets of target genes for Notch and Wnt pathways. Among several available gene sets, we chose the ones having the best differential activity scoring between metastatic and non-metastatic samples for computing Notch and Wnt pathway activities. For computing the p53 pathway activity, we used a set of known p53 primary targets [70] . RNA extraction and quantitative reverse transcription PCR Total RNA from snap-frozen tissue was isolated using trizol extraction (Invitrogen). Extracted RNA (5 μg) was reverse-transcribed with random primers following the manufacturer’s protocol (Invitrogen, superscript). For the quantitative reverse transcription PCR, 100 ng of cDNA was added in a reaction mix containing 0.25 mM of each primer in the LightCycler SybR green master mix (Roche, Diagnostics) with RNase-free water adjusted to a total volume of 20 μl. The PCR programme included a denaturation step at 95 °C for 5 min followed by 40 cycles of 95 °C for 10 s, 60 °C for 30 s and 72 °C for 30 s. All reactions were performed in duplicate in 384-well plates. The quantification was performed using the ΔΔ C t method, by comparing the expression of the target gene in tumour versus normal tissue, relative to the endogenous reference, β 2-microglobulin. Designed and validated primer pairs used are the following pairs: Lgr5 (F) 5′-CAAGCCATGACCTTGGCCCTG-3′ and (R) 5′-TTTCCCAGGGAGTGGATTCTAT-3′; c-Myc : (F) 5′-AAGGCCCCCAAGGTAGTGA-3′ and (R) 5′-TCCAGAAGGGCTTCAATCTG-3′; Ccnd1 : (F) 5′-CCCAACAACTTCCTCTCCTG-3′ and (R) 5′-TCCAGAAGGGCTTCAATCTG-3′; β 2-microglobulin : (F) 5′-GCTATCCAGAAAACCCCTCAAA-3′ and (R) 5′-AGGCGGGTGGAACTGTGTT-3′. Differential expression analysis of EMT genes For EMT gene quantification, we used the mouse EMT ChIP PCR array from Qiagen (84 genes) and used the protocols and analysis recommended by the manufacturer. After filtering out signals of saturated intensity, we obtained gene expression measurements for four tumour and four normal samples. Student’s t -test was performed for each gene to identify significant changes in expression values between tumour and normal samples. Results are represented by histograms of t -scores and P values of the t -tests. We identified 19 genes as being highly differentially expressed between tumour and normal tissue with a fold change of at least 2 and P <0.1. Results obtained for each gene are reported in Supplementary Table 2 . We highlighted the nodes of the map corresponding to the genes analysed in the EMT chip, colouring them according to the t -test values. We used the Fisher’s exact test to assess whether the t -score results obtained for pre-defined gene groups differ from each other. We pre-defined two gene groups, one with genes expected to be upregulated during EMT (Exp-EMT-up) and a second one with genes expected to be downregulated during EMT (Exp-EMT-down). The third group includes all other genes for which we tested the differential expression between tumour samples and normal samples. How to cite this article: Chanrion, M. et al. Concomitant Notch activation and p53 deletion trigger epithelial-to-mesenchymal transition and metastasis in mouse gut. Nat. Commun. 5:5005 doi: 10.1038/ncomms6005 (2014).